A source of the single-stranded DNA substrate for activation-induced deaminase during somatic hypermutation During somatic hypermutation (SHM), activation-induced deaminase (AID) mutates deoxycytidine on single-stranded DNA (ssDNA) generated by the transcription machinery, but the detailed mechanism remains unclear. Here we report a higher abundance of RNA polymerase II (Pol II) at the immunoglobulin heavy-chain variable ( Igh - V ) region compared with the constant region and partially transcribed Igh RNAs, suggesting a slower Pol II progression at Igh - V that could result in some early/premature transcription termination after prolonged pausing/stalling of Pol II. Knocking down RNA–exosome complexes, which could decrease premature transcription termination, leads to decreased SHM. Knocking down Spt5, which can augment premature transcription termination, leads to increase in both, SHM and the abundance of ssDNA substrates. Collectively, our data support the model that, following the reduction of Pol II progression (pausing or stalling) at the Igh-V , additional steps such as premature transcription termination are involved in providing ssDNA substrates for AID during SHM. While antibodies are responsible for the humoral immune response, those antibodies encoded by germline sequences often do not have sufficient affinity or specificity to provide full protection against diverse pathogens. To deal with this, B cells have developed mechanisms to somatically hypermutate (SHM) the V regions of their germline encoded heavy- and light-chain antibody genes. Most mutations are accumulated in the complementarity-determining regions of antibodies to refine their antigen-contacting surfaces. B cells also diversify antibody function by carrying out class switch recombination (CSR), which allows different antigen binding sites to be expressed with different constant regions. Together, SHM and CSR provide us with antibodies that can interact with all antigens, are distributed throughout the body and mediate effective humoral immune protection [1] . Both SHM and CSR require the endogenous mutagenic enzyme activation-induced deaminase (AID) [2] , [3] . As a result of intensive study over the last 13 years, it is now known that AID: (1) deaminates dC to dU and creates point mutations, abasic sites and G:U mismatches [4] ; (2) recruits error-prone DNA repair processes that further contribute to the diversification of mutation spectra by introducing mutations at A/T sites [5] ; (3) requires transcription of the targeted genomic region during both SHM and CSR [6] ; and (4) utilizes single-stranded DNA (ssDNA) as its biochemical substrate [7] . The fact that AID binds and mutates only ssDNA substrates is puzzling because ssDNA is a transient and short-lived form of DNA that is mostly covered by protein complexes during transcription or replication. It is thus unclear exactly how ssDNA is generated and made accessible for AID during SHM or CSR and whether the two different processes share the same mechanism(s). When carrying out SHM and CSR in B cells, AID also occasionally introduces mutations at genomic loci other than antibody genes and these ‘off-target’ mutations are responsible for many B-cell malignancies [8] . Since transcription is necessary for SHM and CSR, AID-mediated mutagenesis must be coordinated with transcriptional machinery [9] . In fact, polymerase II (Pol II) [10] , Spt5 [11] and RNA polymerase associated factor (PAF) [12] have all been reported to interact with AID directly and to affect CSR. However, even though transcription is always accompanied by ssDNA around the synthesis centre of the Pol II complex—the structure referred to as a transcription bubble—the conventional transcription cycle of initiation, elongation and termination is unlikely to supply ssDNA substrates for AID for the following reasons. First, recent structural studies suggest that ssDNA created in the transcription bubble is almost fully covered by either the Pol II complex itself or cofactors like the DRB sensitivity-inducing factor (DSIF, composed of Spt4 and Spt5 proteins) [13] . Such coverage is probably present throughout elongation and even during transcription termination triggered by poly-A signals [14] . Second, whereas transcription initiation involves TFIIH-mediated dsDNA melting at promoter regions before a complete Pol II complex is assembled [15] , AID may be excluded from those regions because a high density of transcription factors normally cover promoters. This is consistent with the fact that AID preferentially targets the immunoglobulin heavy-chain variable ( Igh-V ) coding region but spares regions that are within ~200 bp immediately after the transcription start site (TSS) [4] , [16] , [17] . Nevertheless, several processes accompanying or resulting from transcription have been proposed to help expose ssDNA for AID targeting. These processes include the following: (1) R-loops resulting from special features in the DNA sequence at Igh switch regions but not Igh-V regions [18] , [19] ; (2) negative DNA supercoils occurring at the trailing end of transcription bubbles [20] ; and (3) paused Pol II complexes that are frequently present proximal to the TSS regions [21] . It is noteworthy that pausing only represents one of the three possible states of stalled Pol II complexes and the other two scenarios include backtracking Pol II due to transcription errors and early terminating Pol II due to the failure of error correction [22] . While DNA supercoils generate AID accessible regions on dsDNA plasmids in vitro [23] and paused Pol II complexes play essential roles in CSR [11] , [24] , [25] , the source(s) of ssDNA substrates for AID during SHM of the V region in vivo remains to be established. Premature transcription termination refers to the process when Pol II is released in the middle of a transcribing gene independent of a poly-A termination signal. It is a plausible way of exposing ssDNA around the Pol II catalytic centre for two reasons. First, during premature transcriptional termination, the release of Pol II complex from template DNA may not be coordinated with the transcriptional termination complexes, which could leave the melted dsDNA unprotected. Second, partial transcripts resulting from premature transcription termination negatively regulate Pol II progression specifically around the termination site [26] , which could in turn maintain ssDNA levels at V regions. While detailed mechanisms remain unclear, it is well established that DSIF complex component Spt5 is essential for Pol II processivity since the loss of Spt5 leads to an increase in premature transcription termination in yeast and in mammalian cells [27] , [28] , [29] . On the other hand, a sustained level of existing premature transcription termination requires the RNA exosome through a newly identified feedback mechanism [26] . Based on these considerations, we tested the role of premature transcription termination in SHM by manipulating the levels of Spt5 and the RNA exosome in the mutating human B-cell line, Ramos. Our data suggest that, in addition to Pol II pausing, there is a second set of events like the premature transcription termination process, which B cells may indeed ‘hijack’ to supply ssDNA substrates for AID to mutate at immunoglobulin V regions during SHM. Reduced progression of Pol II at Igh-V region in Ramos cells Since Pol II abundance at specific regions of a transcribing gene is widely used to assess local progression efficiency, we first examined the distribution of Pol II complexes at the actively transcribing Igh -V locus in Ramos cells. The human Burkitt’s lymphoma-derived Ramos cell line has many characteristics of a germinal centre B cell including the constitutive capacity to undergo SHM and a pattern of AID-induced mutations at G:C sites that is similar to what has been observed in vivo [30] . However, analysis of Pol II abundance in wild type Ramos cells is challenging because the size of the hypermutating V region (~400 bp) is at the resolution limit of the chromatin immunoprecipitation (ChIP) analysis. To circumvent this problem, we expanded the AID-targeting region in Ramos by introducing an mCherry fluorescent protein coding sequence into the second exon of the Igh-V locus. Using recombinase-mediated cassette exchange [31] , we replaced the endogenous Ramos V region with an in-frame fusion of the mCherry gene and the endogenous V region ( Fig. 1a ) to provide an ~1.2 kb target for AID as well as a reporter for AID-induced mutations. We confirmed that the entire fusion V exon was able to be targeted by AID-mediated SHM (see below). Using the ChIP assay, we detected on the average ~2–3 times more Pol II at the second exon of Igh-V —the 1.2 kb hypermutating mCherry/ Igh-V fusion region—than at other areas of the gene, that is, the promoter, the downstream intronic enhancer E μ and the constant region ( Fig. 1b ). The relatively higher abundance of Pol II was quite consistent among the different parts of the mCherry/Igh-V fusion (c–f) compared with the relatively lower abundance within the downstream Eμ-Cμ region (h–k) ( Fig. 1c ). This significant but moderate increase in Pol II occupancy in the mCherry/Igh-V region suggested a slowing down of Pol II progression. We also conducted ChIP analysis for Pol II phosphorylated at serine 5 of the carboxy-terminal repeat domain (Pol II S5P), a form of Pol II that is enriched during transcription initiation and gradually decreases throughout elongation. We found that Pol II S5P occupancy stayed high from the promoter region until ~2.5 kb downstream of TSS ( Fig. 1d ). This suggested that Pol II started to transit from initiation phase to elongation phase immediately before E μ. 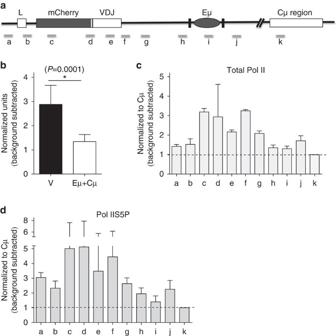Figure 1: Abundance of Pol II complexes at Igh-V region in Ramos cells. (a) The structure of theIgh-Vregion in the reporter Ramos cell line is depicted with grey bars indicating the positions of each primer set used in the following figures and rectangular boxes representing coding exons. (b) ChIP was conducted on reporter cells expressing the AID–ER fusion protein but without 4-OHT treatment using anti-total Pol II, quantified by real-time PCR and normalized to the level at Cμ region after subtraction of immunoglobulin G (IgG) background. Average total Pol II occupancy atIgh-Vregion and downstream regions were compared using student’st-test. (c) The abundance of Pol II at each region shown ina. (d) ChIP was conducted on reporter cells using anti-Pol II S5P and was quantified by real-time PCR. Data were then normalized to signals at the Cμ region after subtraction of IgG background. Data represent the average of two independent experiments and error bars represent s.d. Figure 1: Abundance of Pol II complexes at Igh-V region in Ramos cells. ( a ) The structure of the Igh-V region in the reporter Ramos cell line is depicted with grey bars indicating the positions of each primer set used in the following figures and rectangular boxes representing coding exons. ( b ) ChIP was conducted on reporter cells expressing the AID–ER fusion protein but without 4-OHT treatment using anti-total Pol II, quantified by real-time PCR and normalized to the level at Cμ region after subtraction of immunoglobulin G (IgG) background. Average total Pol II occupancy at Igh-V region and downstream regions were compared using student’s t -test. ( c ) The abundance of Pol II at each region shown in a . ( d ) ChIP was conducted on reporter cells using anti-Pol II S5P and was quantified by real-time PCR. Data were then normalized to signals at the Cμ region after subtraction of IgG background. Data represent the average of two independent experiments and error bars represent s.d. Full size image Spt5 knockdown affects Pol II occupancy and ssDNA patches Reduced progression of Pol II complexes suggested the existence of stalled Pol II at Igh-V regions. Stalled Pol II complexes could represent a paused Pol II, a backtracking Pol II or an early terminating Pol II (ref. 22 ). To address whether the stalled Pol II contributes to SHM and, if so, which of these three processes is responsible, we chose to manipulate the level of the DSIF complex component Spt5. This is because: (1) Spt5 mediates proximal TSS pausing of the RNA polymerase [32] ; and (2) it positively maintains Pol II processivity during elongation [27] , [28] , [29] . Therefore, a decrease in Spt5 level is expected to reduce Pol II pausing but facilitate premature Pol II termination. Of five short hairpin RNA (shRNA) constructs against human Spt5 ( SUPT5H ) tested in Ramos cells, two (#4 and 6) achieved ~50% knockdown at both messenger RNA (mRNA) and protein levels ( Fig. 2a,b , Supplementary Fig. 1 ). Spt5 knockdown (Spt5KD) cells and cells transduced with a control-shRNA (Ctrl-shRNA) expressed similar amounts of steady-state IgH and AID mRNA ( Fig. 2c ). We also found that, as expected, Spt5 abundance at the IgH region was consistently decreased in Spt5KD cells and, to a more variable extent, the total Pol II complex abundance decreased accordingly in two independent experiments ( Fig. 2d ). 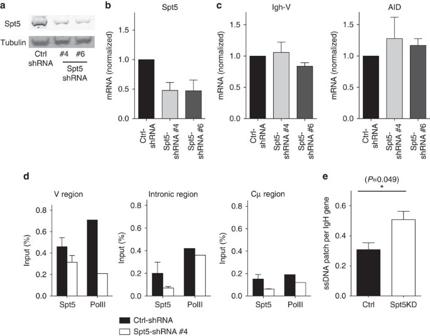Figure 2: Decrease in the cellular Spt5 level is associated with more ssDNA patches. (a) Western blot; and (b) quantitative PCR analysis of Spt5 protein and mRNA level (normalized by cyclophilin B expression) in cells transduced with indicated shRNA(s). (c) Quantitative PCR analysis of mRNA levels of IgH and AID in cells either transduced with Ctrl-shRNA constructs or indicated shRNA against Spt5. (d) ChIP was conducted for Spt 5 and Pol II on cells either transduced with Ctrl-shRNA or shRNA #4 against Spt5 and ChIP products were quantified by quantitative PCR at the indicated region ofIghgene. (e) Abundance of exposed ssDNA patches was quantified using native bisulphite conversion method (see Methods) followed by DNA sequencing. Data represent four independent experiments for part a and two independent experiments for part d (the error bars in this case are the variation in the duplicate PCRs in that experiment wherever applicable). Part b and c represent the average of at least three independent experiments. Part e represents a compiled analysis from two independent experiments usingt-test and error bars represent the s.d. Figure 2: Decrease in the cellular Spt5 level is associated with more ssDNA patches. ( a ) Western blot; and ( b ) quantitative PCR analysis of Spt5 protein and mRNA level (normalized by cyclophilin B expression) in cells transduced with indicated shRNA(s). ( c ) Quantitative PCR analysis of mRNA levels of IgH and AID in cells either transduced with Ctrl-shRNA constructs or indicated shRNA against Spt5. ( d ) ChIP was conducted for Spt 5 and Pol II on cells either transduced with Ctrl-shRNA or shRNA #4 against Spt5 and ChIP products were quantified by quantitative PCR at the indicated region of Igh gene. ( e ) Abundance of exposed ssDNA patches was quantified using native bisulphite conversion method (see Methods) followed by DNA sequencing. Data represent four independent experiments for part a and two independent experiments for part d (the error bars in this case are the variation in the duplicate PCRs in that experiment wherever applicable). Part b and c represent the average of at least three independent experiments. Part e represents a compiled analysis from two independent experiments using t -test and error bars represent the s.d. Full size image Transient patches of ssDNA in chromatin can be detected by treating cross-linked nuclei with bisulphite reagents under non-denaturing conditions [33] , [34] . In this assay, the bisulphite treatment only converts dCs on exposed ssDNA to dUs but cannot convert dCs that are either hybridized with other nucleic acids (dsDNA or RNA:DNA hybrids) or covered by proteins. Using this bisulphite method, we found significantly more non-protected ssDNA patches at the Igh-V region in Spt5KD cells than in Ctrl-shRNA-transduced cells ( Fig. 2e ), suggesting that the decrease in cellular Spt5 levels was associated with more potential AID substrates. Spt5 knockdown is associated with an increase in SHM We first estimated the change of SHM rate on Spt5 reduction in an IgM − Ramos subclone that expressed endogenous levels of AID and had a nonsense mutation in the native V region. We used the IgM gene reversion assay established previously [35] (see Methods) and found that the ~50% reduction in the Spt5 level was accompanied by a significant increase in the SHM rate (5.46 × 10 −5 versus 7.52 × 10 −5 per nucleotide per generation ( P <0.05)) ( Fig. 3a ). 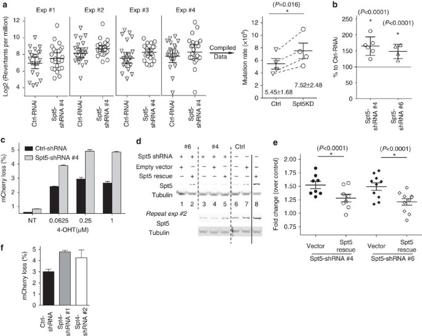Figure 3: Decrease in cellular Spt5 leads to an increase in SHM. (a) Mutation rates of wild type Ramos cells transduced with either Ctrl-shRNA or shRNA #4 against Spt5 were estimated using the reversion assay. In each of the four independent experiments, reversion of 24 clones transduced with either the Ctrl or the #4 Spt5 shRNA was compared (shown in the left panel) and rates of mutation calculated from each experiment were represented by corresponding symbols in the right panel. Statistical analysis was conducted on data compiled from the four independent experiments. (b) Mutation frequency assessed by the reporter cell line as percentage of cells that had lost fluorescence on 4-OHT induction. Data were normalized to Ctrl-shRNA-transduced cells. (c) Indicated amounts of 4-OHT were used to induce AID-mediated mutation as assessed by the loss of fluorescence (NT refers as cells without 4-OHT induction). Data were a representative result of two independent experiments with each condition done in triplicate. (d) An exogenous Spt5 coding construct with partial resistance to shRNA (7 out of 21 nucleotides mutated with no change in amino-acid sequence) was introduced into cells followed by the transduction of indicated shRNA against Spt5. Cells with the exogenous Spt5 rescue construct showed substantial resistance to shRNA-mediated knockdown of Spt5 (lane 2, 5 versus lane 1, 3). Western blots from two independent experiments are shown. Dash and solid lines were used to help distinguish different experimental groups. (e) Restoring the Spt5 level in Spt5KD cells reduced the SHM frequency. (f) Augmented SHM in cells transduced with shRNA against the Spt4 gene. Compiled data are shown ina,b,eandfwith each symbol representing an independent set of experiments. Pairedt-test (a,e) orz-test (b) was used for the statistical analysis and error bars represent the s.d. Representative data of at least two independent experiments were shown inc,d,g. Figure 3: Decrease in cellular Spt5 leads to an increase in SHM. ( a ) Mutation rates of wild type Ramos cells transduced with either Ctrl-shRNA or shRNA #4 against Spt5 were estimated using the reversion assay. In each of the four independent experiments, reversion of 24 clones transduced with either the Ctrl or the #4 Spt5 shRNA was compared (shown in the left panel) and rates of mutation calculated from each experiment were represented by corresponding symbols in the right panel. Statistical analysis was conducted on data compiled from the four independent experiments. ( b ) Mutation frequency assessed by the reporter cell line as percentage of cells that had lost fluorescence on 4-OHT induction. Data were normalized to Ctrl-shRNA-transduced cells. ( c ) Indicated amounts of 4-OHT were used to induce AID-mediated mutation as assessed by the loss of fluorescence (NT refers as cells without 4-OHT induction). Data were a representative result of two independent experiments with each condition done in triplicate. ( d ) An exogenous Spt5 coding construct with partial resistance to shRNA (7 out of 21 nucleotides mutated with no change in amino-acid sequence) was introduced into cells followed by the transduction of indicated shRNA against Spt5. Cells with the exogenous Spt5 rescue construct showed substantial resistance to shRNA-mediated knockdown of Spt5 (lane 2, 5 versus lane 1, 3). Western blots from two independent experiments are shown. Dash and solid lines were used to help distinguish different experimental groups. ( e ) Restoring the Spt5 level in Spt5KD cells reduced the SHM frequency. ( f ) Augmented SHM in cells transduced with shRNA against the Spt4 gene. Compiled data are shown in a , b , e and f with each symbol representing an independent set of experiments. Paired t -test ( a , e ) or z -test ( b ) was used for the statistical analysis and error bars represent the s.d. Representative data of at least two independent experiments were shown in c , d , g . Full size image We then used an independent Ramos cell line (‘reporter line’ described in Fig. 1a and the Methods) that carries the mCherry/VH4–34 fusion at Igh-V locus and expresses AID–ER fusion protein to confirm the effect of knocking down Spt5 on SHM. With this reporter line, the mutation rate can then be quantitatively assessed based on the percentage of cells that lose their fluorescence on 4-hydroxy-tamoxifen (4-OHT) induction of the nuclear localization of AID [36] . Consistent with the reversion assay, ~50–60% more cells lost their fluorescence under the Spt5KD condition than the control cells after 7 days of induction ( Fig. 3b ). While the SHM level reached a plateau with the induction concentration of ~0.25 μM 4-OHT in both Spt5KD and control cells, Spt5KD cells mutated the Igh-V region more efficiently at a lower concentration of inducer (0.0625 μM) than control cells did at the maximum induction level ( Fig. 3c ). These data indicated that the increased level of SHM in Spt5KD cells was not due to the excessive level of active AID molecules in nucleus. Because of the significant increase in the experimental efficiency using the reporter line instead of the reversion assay in analysing the efficiency of SHM, we chose to perform all further mutation analyses on the reporter platform. We next used an shRNA-resistant form (see Methods) of Spt5 to rescue the effect phenotypically. The exogenous Spt5 rescue construct restored Spt5 levels in the knockdown cells close to normal levels (lanes 2 and 5 versus 6 in Fig. 3d , Supplementary Fig. 2 ). Consistent with the regulatory role of Spt5 on SHM, Spt5KD cells (with either the #4 or #6 shRNA construct) significantly reduced their mutation frequencies ( P <0.0001) when cellular Spt5 levels were largely restored ( Fig. 3e ). These data confirmed that the reduced level of Spt5 was the cause of the observed increase in SHM in the Spt5-specific shRNA-transduced cells. Since the DSIF complex is composed of Spt5 and Spt4 molecules, we also tested whether reducing the Spt4 level in cells would have an impact on SHM similar to Spt5KD. Indeed, a similar increase in SHM was observed when endogenous Spt4 level was reduced in the reporter Ramos cells ( Fig. 3f ). Nevertheless, the experiment needs to be interpreted with caution because Spt4 is also a stabilizing factor for Spt5 (ref. 37 ) and the effect of Spt4KD can at least partially be caused by the reduction in the level of general DSIF complexes. Impact of Spt5KD on the characteristics of SHM In the previous section, we used both the reversion of a nonsense mutation in the native Ramos V region and the loss of fluorescence of a reporter in the endogenous Igh-V locus to show that the knockdown of Spt5 resulted in a 50–60% increase in V region mutation. To provide an independent measure of the frequency of mutation per mutated Igh-V gene and to examine the characteristics of the additional mutations, we went on to examine the sequences of the Igh-V fusion genes in mutated Ramos reporter cells by Sanger sequencing. Since in Ramos cells only a small percent of the V regions undergo mutation, we sequenced only those cells that mutated their Igh-V gene sufficiently to cause a loss of fluorescence. Most of the mutations in both the control and the knockdown cells were in AID hot spots. Reduction of Spt5 did not cause a statistically significant change in the distribution of mutations in either the mCherry or the 4–34 part of the fusion V region ( Fig. 4a ). However, the average number of mutations harboured by each mutated Igh-V gene was consistently (but not statistically significantly) increased by about 25% based on three independent experiments ( Fig. 4b ). This provides independent evidence that a decrease in Spt5 leads to not only more V regions being targeted for mutation but also more mutations accumulating in individual mutated Igh-V genes. While these are two different ways of quantifying mutation, the overall impact was estimated by multiplying the ~1.6-fold increase in frequency (based on the fluorescence reporter assay) by the 1.25 increase in mutations per V region, which resulted in a approximately twofold overall increase of AID-induced mutations due to the knockdown of Spt5. The magnitude of this increase is similar to what can be achieved by artificially introducing a termination signal at the immunoglobulin light chain V region in chicken DT40 cells [38] . Spt5 levels did not influence the strand distribution of mutations (mutation preference on the template or the non-template strand) because the incidence of mutations from C or from G was similar (~50%) in both Spt5KD and Ctrl-shRNA-transduced cells ( Fig. 4c ). Interestingly, the frequency of G:C transversions in Spt5KD cells was consistently and significantly higher than control cells ( Fig. 4d ), suggesting that Spt5 might suppress base excision repair or the lack of Spt5 might expose docking sites that facilitate the recruitment of base excision repair machinery. Nevertheless, a difference of UNG recruitment is not likely to be the main reason for our observed increase in SHM upon Spt5 reduction because: (1) UNG mediates only one of the two pathways in the second phase of SHM and accounts for both transversion mutations and error-free repair [4] ; (2) UNG promotes both SHM and CSR while reduction of Spt5 leads to opposite effects on SHM and CSR (see Discussion); and (3) change in the availability of UNG does not influence overall mutation frequency [39] . Hence, the increase of the overall SHM rate most likely resulted from the initial increase of the frequency of deamination. Overall, these data suggest that reduction in the Spt5 level promotes SHM in a general manner without any spatial preference. 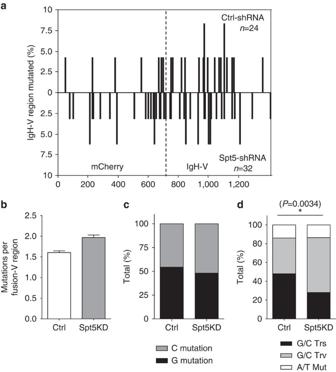Figure 4: Impact of Spt5KD on the characteristics of SHM. (a) Distribution of mutations in the fusion V region (seeFig. 1) from cells either transduced with Ctrl-shRNA or shRNA against Spt5 was analysed by SHMTool (http://scb.aecom.yu.edu/cgi-bin/p1). The illustrated distribution is calculated from one representative sequencing experiment. The vertical dashed line at 720 bp marks the border between the mCherry and endogenous 4–34 V regions. (b) Mutations perIgh-Vgene, (c) G or C mutation frequency and (d) mutation types were summarized in indicated cell types from two independent sequencing experiments. In total, 45Igh-Vsequences were sequenced for Ctrl-shRNA-transduced cells and 54 for Spt5KD cells. Two by two contingency table analysis was used for statistical analysis inb,c,d. Figure 4: Impact of Spt5KD on the characteristics of SHM. ( a ) Distribution of mutations in the fusion V region (see Fig. 1 ) from cells either transduced with Ctrl-shRNA or shRNA against Spt5 was analysed by SHMTool ( http://scb.aecom.yu.edu/cgi-bin/p1 ). The illustrated distribution is calculated from one representative sequencing experiment. The vertical dashed line at 720 bp marks the border between the mCherry and endogenous 4–34 V regions. ( b ) Mutations per Igh-V gene, ( c ) G or C mutation frequency and ( d ) mutation types were summarized in indicated cell types from two independent sequencing experiments. In total, 45 Igh-V sequences were sequenced for Ctrl-shRNA-transduced cells and 54 for Spt5KD cells. Two by two contingency table analysis was used for statistical analysis in b , c , d . Full size image RNA exosome and premature transcription termination in SHM The finding that a decrease in Spt5 levels is accompanied by an increase in the rate of SHM suggested that premature transcription termination might be associated with and could contribute to SHM. To explore this possibility further, we knocked down the RNA–exosome complex because: (1) the RNA exosome helps to induce premature termination of transcription [26] ; and (2) the exosome core components facilitate SHM in a biochemical assay [40] in vitro , although this has not been established in vivo . The RNA–exosome complex is composed of two ribonuclease units and a nine sub-unit core including Rrp40 ( EXOSC3 ) [41] , [42] , a molecule that has a profound impact in AID-mediated mutation activity in vitro [40] . Therefore, we tested the role of Rrp40 in SHM using Ramos cells. The maximum reduction we achieved from five shRNAs against the exosome core component Rrp40 was ~30% at mRNA level ( Fig. 5a ). This is probably because an extensive decrease in its level is cytotoxic considering the essential role of RNA exosome for ribosomal RNA processing [43] . However, based on data from two independent shRNA constructs, this small decrease of Rrp40 level was sufficient to reduce the frequency of SHM by ~30–40% ( P <0.05) ( Fig. 5b ). The Rrp40 knockdown did not significantly change the overall distribution of mutations in either the mCherry or the endogenous V region ( Fig. 5c ). In addition, there was no increase in the numbers of mutations on the non-template strand compared with the template strand ( Fig. 5d ), nor did we find any change in mutation pattern resulting from the reduced Rrp40 level ( Fig. 5e ). This indicated that the RNA–exosome complexes could promote SHM in a general way rather than solely through the suggested nascent RNA degradation mechanism that would help to preferentially expose template ssDNA [40] . Our data, however, cannot rule out the possibility that the latter mechanism may also play an important role in SHM because our limited ability to reduce RNA–exosome levels might have precluded us from observing such an effect. 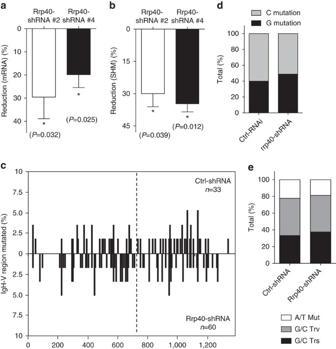Figure 5: RNA exosome and SHM. (a) Knockdown efficiency of Rrp40 was assessed by quantitative PCR and percentage of reduction was calculated by comparing with Ctrl-shRNA-transduced cells. (b) SHM rate was assessed in Rrp40 knockdown cells and Ctrl-shRNA-transduced cells in the Ramos reporter cells and the reduction of SHM level was calculated accordingly. Combined data from three independent experiments were used to detect significant reduction associated with a reduced level of cellular Rrp40. (c) Distribution of mutations in cells either transduced with Ctrl-shRNA or shRNA against Rrp40 were analysed by SHMTool. Data represent the compiled analysis from two independent sequencing experiments. (d) G or C mutation frequency and (e) mutation type were summarized in cells under the indicated conditions. A total of 33Igh-Vsequences were sequenced from Ctrl-shRNA-transduced cells and 60 from Rrp40KD cells. A compiled analysis of three independent experiments was conducted ina,busingt-test and error bars represent the s.d. Two by two contingency table analysis was used for statistical analysis ind,e. Figure 5: RNA exosome and SHM. ( a ) Knockdown efficiency of Rrp40 was assessed by quantitative PCR and percentage of reduction was calculated by comparing with Ctrl-shRNA-transduced cells. ( b ) SHM rate was assessed in Rrp40 knockdown cells and Ctrl-shRNA-transduced cells in the Ramos reporter cells and the reduction of SHM level was calculated accordingly. Combined data from three independent experiments were used to detect significant reduction associated with a reduced level of cellular Rrp40. ( c ) Distribution of mutations in cells either transduced with Ctrl-shRNA or shRNA against Rrp40 were analysed by SHMTool. Data represent the compiled analysis from two independent sequencing experiments. ( d ) G or C mutation frequency and ( e ) mutation type were summarized in cells under the indicated conditions. A total of 33 Igh-V sequences were sequenced from Ctrl-shRNA-transduced cells and 60 from Rrp40KD cells. A compiled analysis of three independent experiments was conducted in a , b using t -test and error bars represent the s.d. Two by two contingency table analysis was used for statistical analysis in d , e . Full size image Premature transcription termination likely occurs at Igh-V Overall, our experiments confirmed the positive role of RNA exosome core component Rrp40 in optimal SHM. Together with the observed increase in SHM on Spt5 reduction, they provided strong support for a positive role of premature transcription termination in SHM. We therefore tested whether premature transcription termination events happened on the Igh gene. Early transcription termination events should result in a higher abundance of transcripts containing only the 5′ end of the gene compared with transcripts containing both 5′ and 3′ ends. Such an imbalance could serve as a surrogate indicator for premature transcription termination and could be estimated by quantifying the absolute copy number of RNA transcripts containing various portions of the gene in total RNA. To do this, we constructed a plasmid harbouring a single copy of each region to be investigated. Using this plasmid and real time quantitative PCR, we generated individual standard curves of the copy numbers (estimated by the molecular weight of the plasmid) against the Ct (cycle threshold) values for each region of interest. These standard curves were then used to determine the absolute quantity of RNA transcripts containing the designated region in total RNA. This quantification method worked effectively, as exemplified by its ability to distinguish the intron region f because of its low abundance (~2–4%) compared with the mature full-length Igh mRNA ( Fig. 6a ). In support of our hypothesis, we observed approximately two fold more RNA transcripts containing the Igh variable region ( Igh-V fusion) than those containing the constant region (Cμ) in Ramos cells ( Fig. 6a ) when cDNAs were synthesized using random hexamers. Partial Igh transcripts containing only the 5′ end of the Igh gene were not polyadenylated ( Fig. 6b ) since this bias was not observed when cDNAs were synthesized using poly-T oligonucleotides (the lower signals detected at the 5′ end of the mRNA compared with the constant region were likely due to the limitation in the enzymatic processivity of the reverse transcriptases). Consistent with the important role of RNA exosome in premature transcription termination, the reduction in Rrp40 levels reduced the bias of higher 5′ only transcripts over the full-length mRNA ( Fig. 6c ). These findings suggest that premature transcription termination does occur naturally at the Igh-V region with its level positively correlating with SHM in B cells. 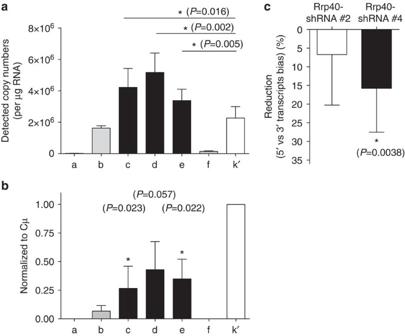Figure 6: Premature transcription termination likely occurs at Igh-V region. (a) Absolute quantification of transcript abundance containing each indicated gene region was conducted by real-time PCR using the corresponding primer sets. Ct value was used to calculate the copy number from a standard curve generated in parallel using the control plasmid template (see Experimental Procedures). Data represent the average of four independent experiments (error bar represents s.d.) and pairedt-test is used in statistical analysis. (b) RNA quantification analysis similar to that in part a was performed on cDNA from poly-T-mediated reverse transcription templates. Data represent the average of three independent experiments.T-test was employed to detect any significant reduction. (c) The bias of abundance in transcripts containing only 5′ end versus full-length were computed as a ratio of the copy number containing 5′ coding region over transcripts containing Cμ from either Rrp40 knockdown cells or Ctrl-shRNA-transduced cells. The reduction of bias was then calculated by comparing Rrp40KD cells to Ctrl-shRNA-transduced cells. Data represented the average of all three regions detected by quantitative PCR at the second exon ofIghgene (regions c, d, e indicated inFig. 1a) from three independent experiments.a,brepresent a compiled analysis of three independent experiments with error bars representing the s.d. Figure 6: Premature transcription termination likely occurs at Igh-V region. ( a ) Absolute quantification of transcript abundance containing each indicated gene region was conducted by real-time PCR using the corresponding primer sets. Ct value was used to calculate the copy number from a standard curve generated in parallel using the control plasmid template (see Experimental Procedures). Data represent the average of four independent experiments (error bar represents s.d.) and paired t -test is used in statistical analysis. ( b ) RNA quantification analysis similar to that in part a was performed on cDNA from poly-T-mediated reverse transcription templates. Data represent the average of three independent experiments. T -test was employed to detect any significant reduction. ( c ) The bias of abundance in transcripts containing only 5′ end versus full-length were computed as a ratio of the copy number containing 5′ coding region over transcripts containing Cμ from either Rrp40 knockdown cells or Ctrl-shRNA-transduced cells. The reduction of bias was then calculated by comparing Rrp40KD cells to Ctrl-shRNA-transduced cells. Data represented the average of all three regions detected by quantitative PCR at the second exon of Igh gene (regions c, d, e indicated in Fig. 1a ) from three independent experiments. a , b represent a compiled analysis of three independent experiments with error bars representing the s.d. Full size image As Spt5 is essential for optimal CSR [11] , [44] and interacts with AID [11] , it is surprising that a reduction in Spt5 levels facilitates SHM. However, this discrepancy can be an indication of the distinct sources of ssDNA substrates for AID during SHM and CSR. Whereas R-loops are the major source of ssDNA during CSR, we propose here (see Fig. 7 ) that premature transcription termination provides ssDNA substrates for AID during SHM. Since mutation rates exceeding 10 −3 per base per generation will introduce too many nonsense mutations for efficient affinity maturation [45] , the complex role of Spt5 in SHM may have evolved to achieve optimal antibody diversification. Moreover, it is noteworthy that Spt5 seems to also influence the non-homologous end joining and homologous recombination processes [44] , both of which are important for CSR but largely dispensable for SHM. Thus, dissimilar roles of Spt5 in SHM and CSR probably reflect the distinct molecular mechanisms involved in these two processes. 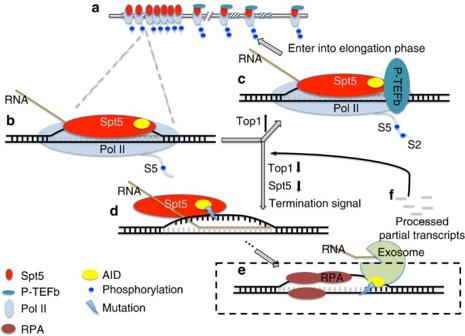Figure 7: Model of the premature transcription termination as a source of ssDNA AID substrates. The progression of Pol II reduces at the mutatingIgh-Vregion, which leads to accumulation of stalling Pol II complexes (a,b). Most stalled Pol II complexes return to elongation after Pol II co-factor Spt5 recruits P-TEFb complexes that release pausing by phosphorylating C-terminal domains of both Spt5 and Pol II (c). However, non-resolvable pausing occurs stochastically, leading to premature transcription termination. Those early terminated Pol II complexes leave the unwound DNA region open with non-template ssDNA strand ready for AID targeting immediately (d). RPA complexes are then recruited to cover exposed non-template ssDNA while RNA:DNA hybrids are processed likely through nascent RNA removal process of transcription termination, which leaves single-strand template DNA sensitive to AID (e). Partial transcripts are processed by the exosome complex, likely providing short RNA to in turn reduce Pol II progression atIgh-Vand sustain the premature termination level there (f). Figure 7: Model of the premature transcription termination as a source of ssDNA AID substrates. The progression of Pol II reduces at the mutating Igh-V region, which leads to accumulation of stalling Pol II complexes ( a , b ). Most stalled Pol II complexes return to elongation after Pol II co-factor Spt5 recruits P-TEFb complexes that release pausing by phosphorylating C-terminal domains of both Spt5 and Pol II ( c ). However, non-resolvable pausing occurs stochastically, leading to premature transcription termination. Those early terminated Pol II complexes leave the unwound DNA region open with non-template ssDNA strand ready for AID targeting immediately ( d ). RPA complexes are then recruited to cover exposed non-template ssDNA while RNA:DNA hybrids are processed likely through nascent RNA removal process of transcription termination, which leaves single-strand template DNA sensitive to AID ( e ). Partial transcripts are processed by the exosome complex, likely providing short RNA to in turn reduce Pol II progression at Igh-V and sustain the premature termination level there ( f ). Full size image Genome-wide Pol II occupancy studies have revealed a large number of genes with stalled Pol II complexes in the transcribing regions. Although the fate of these stalled Pol II complexes remains under debate, one possibility among several others (like pausing or stalling), is that at least some of them will eventually lose all processivity and terminate transcription prematurely [21] , [22] . Our RNA transcript analysis identified partially transcribed Igh genes in B cells ( Fig. 6 ). Although a bias towards 5′ region containing transcripts could result from preferential 3′ degradation of mRNA, it more likely reflects a role of premature transcription termination in SHM since: (1) Pol II is enriched in Igh-V region at a similar level as that reported around transcription termination sites ( Fig. 1 ) [21] , [22] ; (2) a reduction in Spt5 leads to an increase in SHM and in the frequency of ssDNA patches at Igh-V region ( Figs 2e and 3 ); (3) the RNA exosome is required for optimal SHM ( Fig. 5 ); and (4) insertion of a transcription termination signal at the Igh-V region in DT40 cells results in increases of both Pol II accumulation and SHM upstream of the termination signal [38] . Together these findings support the idea that premature transcription termination contributes to SHM by supplying ssDNA substrates for AID. This premature transcription termination at the Igh-V region could be the consequence of frequent stalling (slow progression) and the stochastic loss of Pol II processivity physiologically, which could expose unwound DNA templates for AID to mediate SHM ( Fig. 7 ). Consistent with this idea, NEDD4, an E3-ubiquitinase that can mediate the degradation of unresolvable stalling Pol II, has been found at AID-targeted regions during CSR [46] . This confirms that Pol II complexes can indeed ‘leave’ their template in the middle of transcriptional process, which may provide AID access to the single-stranded transcription bubble. Interestingly, this model is also consistent with the observation that hypermutating dark zone germinal centre B cells actually reduce their surface Ig level and that could be due to an increase in premature transcription termination at hypermutating V regions [47] . Two different processes have recently been proposed to provide ssDNA substrates for AID. First, paused Pol II complexes correlated with the generation of R-loop structures at IgH switch regions, which positively contributes to CSR [18] , [19] . If paused Pol II complexes themselves are also sufficient to facilitate SHM, the reduction in DSIF (Spt5/Spt4 complex) level should lead to a decrease in both Pol II pausing and SHM. On the contrary, we observed an increase in SHM when the Spt5 level was reduced in Ramos B cells. Since the reduction of cellular Spt5 is known to decrease Pol II processivity and hence promote premature transcription termination [27] , [28] , [29] , these observations suggested that premature transcription termination could be playing an important role in SHM. Second, accumulation of DNA supercoils around the transcribing Pol II complex has also been proposed as a source of AID substrates [23] , [34] . AID can mutate supercoiled DNA in vitro and reduction of the DNA supercoil relieving factor topoisomerase I results in an increase in SHM [48] . However, supercoiled DNA should expose both strands of a DNA molecule symmetrically, but this remains to be examined by the ssDNA patch analysis by deeper sequencing for the V region in vivo [33] , [34] . Our model ( Fig. 7 ) of the premature transcription termination process as a source of ssDNA for AID during SHM suggests that: (1) the hypersensitive mutation region is similar to the size of a transcription bubble (14–18 bp); (2) any factors that reduce Pol II processivity such as a decreased level of elongation factors or increased abnormal DNA structures like supercoils will facilitate SHM [48] ; (3) an artificial increase of Pol II complex termination by adding termination signals at V region promotes SHM [38] ; and (4) template and non-template ssDNA are not likely exposed to AID simultaneously. We also ( Fig. 7 ) hypothesize that on premature termination, unwound non-template ssDNA is exposed while template strand may remain hybridized with nascent RNA. Later, non-template ssDNA in the transcription bubble gets protected by RPA while RNA:DNA hybrids in the same transcription bubble will be processed through an RNA removal mechanism during termination [49] to expose the template strand ssDNA for AID to target. Such sequential exposure of ssDNA for AID targeting is probably important for keeping the frequency of DNA double-strand breaks low (<~10%) at the Igh-V regions during SHM [30] . How AID targets Ig loci with high specificity in B cells remains a central question in B-cell biology. Although our data indicate that the frequency of AID substrates strongly influences the mutation frequency in a SHM-competent cell, the occurrence of ssDNA at the Igh-V region is probably not sufficient for eliciting the SHM process. In fact, the premature transcription termination process is likely to be determined by DNA elements independent of AID and SHM. This notion is consistent with recent observations that neither the accumulation of Pol II at the switch regions [24] nor the ssDNA frequency [33] at Igh-V region is dependent on AID. Moreover, the level of Pol II accumulation at the Ig-L locus in DT40 cells is independent of either the surrounding cis-elements capable of promoting SHM or the presence of AID [50] . Thus, although we have elucidated a novel mechanism utilized by B cells to provide ssDNA substrate for AID during SHM, the susceptibility of the variable region to SHM and the specificity of AID targeting to those regions in B cells are probably subject to several more levels of control rather than a simple interaction of the enzyme and its substrates. It is however interesting to investigate in the future what source(s) of ssDNA is used in off-target mutation sites of AID and whether they share similar mechanisms with the Igh-V region. Cell lines and antibodies The wild type human Burkitt’s lymphoma cell line Ramos has been described in refs 30 , 35 . The modified reporter Ramos cell line was established by replacing the endogenous 4–34 Igh-V region with mCherry-4–34 fusion fragment ( Fig. 1a ) using recombinase-mediated cassette change. Briefly, a LoxP-flanked hygromycin resistance gene was integrated into endogenous Igh-V locus by homologous recombination. The mCherry reporter cassette was then knocked into the Igh-V locus through Cre-mediated recombination [31] . The Ramos clone used to construct this reporter line was preselected to have an undetectable level of AID protein and confirmed not to undergo SHM. Cells containing mCherry– Igh-V fusion were then transfected with AID–ER fusion protein [36] and clones were selected based on their capacity for undergoing SHM in a 4-OHT (Sigma-Aldrich)-inducible manner. Cells were considered to have undergone SHM when they reduced their mCherry fluorescence based on flow cytometry analysis. Antibodies used in this study were anti-Pol II C-terminal repeats (Abcam), anti-Pol II C-terminal repeats (serine 5 phosphorylated) (Abcam), anti-Spt5 (Santa Cruz) (1:250 dilution), anti-tubulin (Sigma-Aldrich) (1:2,500 dilution). Real-time PCR quantification In ChIP experiments, ChIP DNA precipitated with a specific antibody (1 μg per reaction) was analysed with the ΔΔCt method using SYBR Green PCR Master Mix (Life Technologies or KAPA Biosystems) and was normalized to input DNA. PCR efficiency was estimated using serial dilutions and the signal was adjusted accordingly. In all experiments, rabbit anti-rat polyclonal antibody was used as the negative control and the ChIP signal from it was subtracted from each sample before further analysis. For absolute quantification of RNA transcripts, a single plasmid containing a single copy of each region of interest was made and the copy number was estimated using the molecular weight calculated based on the size of the plasmid. The plasmid was then used as a standard in the standard curve method of quantitative PCR and the copy number was calculated by ViiA 7 real-time PCR software (Life Technologies). Primers used in the study are listed in Supplementary Table 1 . Lentiviral transduction and shRNA Lentiviral particles containing designated shRNA were prepared by shRNA Core Facility at Albert Einstein College of Medicine. All the shRNA constructs were obtained from the human TRC Library (Thermo Scientific) with sequences listed in Supplementary Table 2 . Control-shRNA (Ctrl-shRNA) is the SHC002 construct from Sigma-Aldrich. Ramos cells were transduced with ~3:1 multiplicity of infection and were subjected to Puromycin (Gibco, Life Technology) selection for 7–9 days. Successful knockdown of targeted genes was verified by real-time PCR and in the case of Spt5, western analysis as well. An shRNA-resistant form of human Spt5 was created by replacing 7 of the 21 nucleotides of the shRNA-targeting sequence but keeping amino-acid sequence untouched. Mutation analysis To obtain the mutation pattern, cells that had lost their mCherry fluorescence were sorted by flow cytometry to extract their genomic DNA (Qiagen). The mCherry– Igh-V fusion region was amplified using PfuTurbo (Agilent) cloned into the sequencing vector and Sanger sequenced in both directions to cover the whole ~1.3 kb region. Sequencing data were then aligned by ClustalW2 and analysed using SHMTool. ssDNA detection by Bisulphite treatment In situ bisulphite treatment of cross-linked cellular nuclei under non-denaturing conditions was conducted to detect ssDNA patches that were natively exposed in chromatin [33] , [34] . The final concentration of bisulphite was reduced to ~2 M to improve DNA recovery and a new KAPA HiFi Uracil+ kit (KAPA Biosystems) was used in the DNA amplification step to improve the accuracy of the analysis. The whole fusion of mCherry and Ramos Igh-V was amplified, cloned into vector and sequenced by Sanger sequencing. Estimation of mutation rate by IgM reversion assay Individual clones of IgM-negative Ramos cells expressing the endogenous VH4–34 heavy-chain V region bearing a stop-codon [35] were allowed to accumulate mutations for 3 weeks. Any mutations that change the stop-codon into a sense codon will allow its descendants to become IgM positive. The frequency of those reverted cells was examined by flow cytometry. After analysing sufficient numbers of clones, a mutation rate at that specific site could be estimated by maximal likelihood method [51] . Statistical analysis All statistical analyses were conducted using Prism 6 software. Throughout the data, * represented that the statistical significance was achieved and P -value was illustrated correspondingly. Error bars represent s.d. among independent experiments. In the cases where multiple experiments were compiled together, a paired Student’s t -test was used. How to cite this article : Wang, X. et al . A source of the single-stranded DNA substrate for activation-induced deaminase during somatic hypermutation. Nat. Commun. 5:4137 doi: 10.1038/ncomms5137 (2014). The funders had no role in study design, data collection and analysis, decision to publish or preparation of the manuscript.